Equilibrium selectivity alone does not create K+-selective ion conduction in K+channels Potassium (K + ) channels are selective for K + over Na + ions during their transport across membranes. We and others have previously shown that tetrameric K + channels are primarily occupied by K + ions in their selectivity filters under physiological conditions, demonstrating the channel’s intrinsic equilibrium preference for K + ions. Based on this observation, we hypothesize that the preference for K + ions over Na + ions in the filter determines its selectivity during ion conduction. Here, we ask whether non-selective cation channels, which share an overall structure and similar individual ion-binding sites with K + channels, have an ion preference at equilibrium. The variants of the non-selective Bacillus cereus NaK cation channel we examine are all selective for K + over Na + ions at equilibrium. Thus, the detailed architecture of the K + channel selectivity filter, and not only its equilibrium ion preference, is fundamental to the generation of selectivity during ion conduction. Ion channels are essential to maintain ionic homoeostasis in cells and to support rapid cellular signalling. Tetrameric cation channels facilitate the flow of Na + , K + and Ca 2+ ions across cellular membranes. These channels have two essential functional properties – they selectively conduct specific ions and they gate open/closed in response to stimuli [1] . Although channel selectivity has been studied for decades, fundamental questions remain about how a K + channel is able to conduct K + ions ( r =1.33 Å) rapidly while selecting against the slightly smaller Na + ion ( r =0.98 Å). For example, is a difference between the equilibrium affinities for K + ions over Na + ions sufficient to explain K + selectivity during conduction as some models suggest [2] ? Because equilibrium affinity is a thermodynamic parameter, it captures many different physical–chemical determinants of ion selectivity in one quantitative term. If an equilibrium preference is insufficient to explain selectivity, then what kinetic barriers are needed [2] ? A variety of experimental techniques all support the conclusion that different K + channels have a preference for K + ions over Na + ions at equilibrium [3] , [4] , [5] , [6] , [7] , [8] , [9] , [10] , [11] , [12] , [13] , [14] , [15] , [16] , [17] , [18] , [19] , [20] , [21] . The simplest mechanism to explain ion selectivity is that the equilibrium preference of a channel determines its selectivity during ion conduction. The recent crystal structures and functional data on the non-selective Bacillus cereus NaK channel and its mutants provide a unique opportunity to test this hypothesis [22] , [23] . The NaK channel has the same overall architecture as K + channels but has a selectivity filter formed from the sequence TVGDG instead of the canonical TVGYG sequence found in most K + channels ( Fig. 1c ) [24] , [25] . The K + channels contain four contiguous K + ion-binding sites in their selectivity filter, but in the NaK filter the two outermost sites (S1 and S2 of K + channels) are replaced with a water-containing vestibule. As a result, only the contiguous S3 and S4 sites remain of the filter. Mutations in the selectivity filter of the NaK channel transform it into channels with two, three or four contiguous sites ( Fig. 1 ) [22] , [23] . Remarkably, the channel with four contiguous sites selectively conducts K + ions, whereas channels with two or three sites remain non-selective. 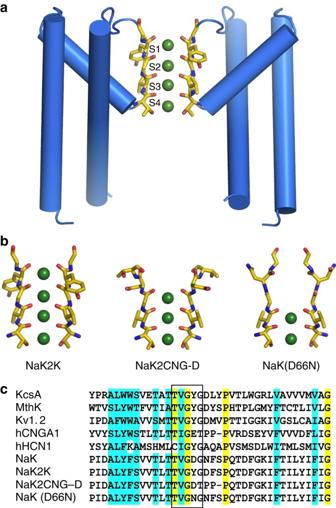Figure 1: Structure of a K+channel and the selectivity filter of mutant NaK channels. (a) A cartoon diagram of the MthK channel (pdb 2LDC) showing two of the four subunits in blue. (b) A comparison of the number of K+binding sites in the selectivity filter of NaK2K, NaK2CNG-D and NaK(D66N) channels. The selectivity filters are yellow sticks and K+ion-binding sites are indicated with a green sphere. (c) A sequence alignment of the selectivity filter for various tetrameric cation and mutant NaK channels used in this study. The box indicates the region shown in panelb. Figure 1: Structure of a K + channel and the selectivity filter of mutant NaK channels. ( a ) A cartoon diagram of the MthK channel (pdb 2LDC) showing two of the four subunits in blue. ( b ) A comparison of the number of K + binding sites in the selectivity filter of NaK2K, NaK2CNG-D and NaK(D66N) channels. The selectivity filters are yellow sticks and K + ion-binding sites are indicated with a green sphere. ( c ) A sequence alignment of the selectivity filter for various tetrameric cation and mutant NaK channels used in this study. The box indicates the region shown in panel b . Full size image Is the equilibrium selectivity sufficient to explain ion selectivity during conduction? Here, we address this question by employing isothermal titration calorimetry (ITC) to measure the equilibrium properties of non-selective and K + -selective mutant NaK channels. We use electrophysiology to characterize the selectivity properties of mutant NaK channels during ion conduction. Previous ITC-based experiments on the KcsA and MthK K + channels revealed a strong preference for K + ions over Na + ions at equilibrium [20] , [21] . If equilibrium selectivity alone is sufficient to explain selective ion permeation of a channel, then the four-site mutant NaK channel should also have a K + preference at equilibrium, whereas the two- and three-site mutant NaK channels should be non-selective at equilibrium. We found that the non-selective channels are all highly selective for K + over Na + ions at equilibrium, demonstrating that equilibrium selectivity alone cannot explain ion conduction selectivity. We conclude that the selectivity of K + channels is based on a mechanism that requires multiple K + ions to bind selectively and simultaneously in the channel’s filter, whereas this mechanism is disrupted in the non-selective channels. Ion selectivity in the four-site NaK2K channel We used mutant NaK channels to understand the ion selectivity properties of K + channels. It was therefore essential to determine whether mutant NaK channels can have the physical and functional properties of natural K + channels. A central feature of all K + channels is that they selectively conduct K + ions through a selectivity filter that contains four contiguous ion-binding sites, with adjacent sites sharing ligand-binding oxygen atoms ( Fig. 1a ) [8] , [11] , [26] , [27] , [28] , [29] . The NaK2K mutant channel, which contains four ion-binding sites, was previously shown in a high-resolution crystal structure to have a selectivity filter indistinguishable from other K + channels ( Fig. 1b ) [22] . We measured the ion permeability ratio in mixed-ion conditions using purified NaK2K channels reconstituted into liposomes to allow Na + and K + ions to directly compete for binding to the selectivity filter ( Fig. 2a ). Single-channel recordings using a vertical bilayer system were obtained with 50 mM KCl and 150 mM NaCl in the cup and 200 mM KCl in the chamber. In these conditions, NaK2K has a reversal potential of −32±3 mV (mean±s.d., n =6), which corresponds to a permeability ratio of 21 (K + :Na + ); a non-selective channel would reverse near 0 mV and a perfectly K + -selective channel would reverse at −35 mV. A similar permeability ratio of ~25 was obtained using bi-ionic conditions in giant liposome patches [22] . NaK2K, like natural K + channels, is selective for K + over Na + during ion conduction. 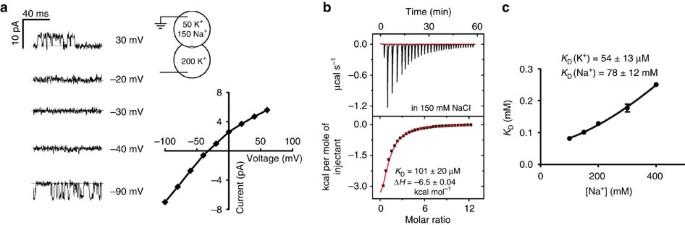Figure 2: Ion binding and permeation of NaK2K channel. (a) Single-channel traces at different membrane potentials (left) and theI–Vcurve (right). Currents are recorded with 150 mM NaCl+50 mM KCl in the cup (outside) and 200 mM KCl in the chamber (inside). The dotted lines mark the closed, zero current level. (b) Thermogram of K+binding to NaK2K in the presence of 150 mM NaCl (top). The integrated heat exchange from each injection is fit to a binding isotherm to obtain the relevant thermodynamic parameters (bottom). (c) The apparent affinity of K+ions for NaK2K as a function of NaCl concentration in solution. The line shows the fit to a competition binding equation described in the methods to obtainKD(K+) andKD(Na+); the mean of three or more experiments and their s.e.m. are plotted. Figure 2: Ion binding and permeation of NaK2K channel. ( a ) Single-channel traces at different membrane potentials (left) and the I – V curve (right). Currents are recorded with 150 mM NaCl+50 mM KCl in the cup (outside) and 200 mM KCl in the chamber (inside). The dotted lines mark the closed, zero current level. ( b ) Thermogram of K + binding to NaK2K in the presence of 150 mM NaCl (top). The integrated heat exchange from each injection is fit to a binding isotherm to obtain the relevant thermodynamic parameters (bottom). ( c ) The apparent affinity of K + ions for NaK2K as a function of NaCl concentration in solution. The line shows the fit to a competition binding equation described in the methods to obtain K D (K + ) and K D (Na + ); the mean of three or more experiments and their s.e.m. are plotted. Full size image Equilibrium affinity measurements of the KcsA and MthK K + channels revealed that they are selective for K + during ion conduction and bind K + ions selectively at equilibrium [20] . It was therefore of interest to determine whether the NaK2K channel also selectively binds K + over Na + ions at equilibrium. ITC quantifies the heat change upon ligand binding to a protein, and is used to measure the equilibrium binding affinities between ions and transport proteins [21] , [30] . A thermogram of K + binding to NaK2K solubilized in detergent is shown in Fig. 2b . The data are fit to a one-site binding model to give the total enthalpy of the reaction and the binding affinity ( Fig. 2b ). Although K + channels have more than one ion in their selectivity filter during ion conduction, the data fit well to either a one or two ion-binding model. It is unclear why we do not observe two distinct ion-binding events, but a possible explanation is that both ions bind with similar affinity and enthalpy. This would make the individual binding events inseparable at the resolution of these experiments and the measured affinity would represent a combination of the individual ion-binding events. As expected based on the similar physical and functional characteristics of the NaK2K channel and K + channels, NaK2K is selective for K + at equilibrium. The affinity for K + ions is in line with the observed values for other K + channels [20] , [21] . The results suggest that NaK2K is selective for K + at equilibrium because K + ions are able to outcompete the much more abundant Na + ions in the buffer. The ion selectivity at equilibrium was determined by measuring the apparent K + affinity in the presence of different concentrations of Na + . This competition mimics the competition encountered within the channel during ion conduction, when ion selectivity is calculated by measuring the reversal potential of mixed-ion conditions. Figure 2c is a plot of the apparent affinity of K + as a function of Na + ion concentration, and those data are fit to the competition model described in Methods. The affinity of NaK2K for K + is 54 μM and that of Na + is 78 mM, which is a ~1,500-fold selectivity of K + over Na + at equilibrium ( Table 1 ). A Hill coefficient ( n ) of 1.4±0.3 is calculated that may originate from interactions between ions within the filter. In addition, K + ions prefer to reside within the oxygen cage of the selectivity filter, whereas Na + ions are found both within the oxygen cage and in the plane of the atoms forming the cage [9] , [11] , [21] , [31] . This difference in binding-site preferences within the selectivity filter could result in a non-stoichiometric displacement of Na + for K + ions, which was also seen in KcsA and MthK channels [20] . Collectively, these results mean that the K + -selective NaK2K channel retains the same basic equilibrium selectivity properties found in K + channels studied to date, demonstrating that the mutant NaK channels can be profitably used to study K + channel selectivity. Table 1 Thermodynamic parameters for Na + and K + ions binding to mutant NaK channels. Full size table Ion selectivity in the three-site NaK2CNG-D channel We next examined the NaK2CNG-D mutant of NaK, which was originally constructed to mimic the selectivity filter of the cyclic-nucleotide-gated (CNG) channels [23] . Its selectivity filter is comprised of three contiguous ion-binding sites that are very similar to the S2–S4 K + binding sites in K + channels ( Fig. 1b ). Like CNG channels, NaK2CNG-D is non-selective for K + and Na + during ion conduction when measured in either mixed-ion or bi-ionic conditions. A permeability ratio of 1.4±0.2 (K + :Na + ; mean±s.d., n =3) in mixed-ion condition was measured ( Fig. 3a ), confirming the lack of selectivity observed in bi-ionic conditions [22] . If equilibrium ion selectivity is a major determinant of selectivity during ion conduction, then NaK2CNG-D should be non-selective at equilibrium. 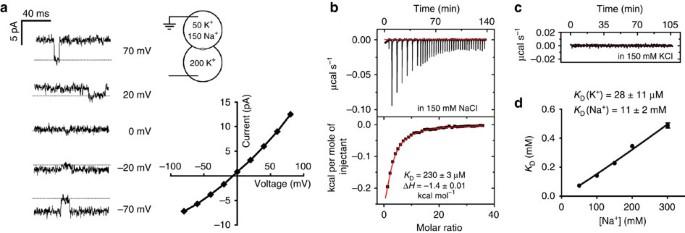Figure 3: Ion binding and permeation of NaK2CNG-D. (a) Single-channel traces at different membrane potentials (left) and theI–Vcurve (right). Currents are recorded with 150 mM NaCl+50 mM KCl in the cup (outside) and 200 mM KCl in the chamber (inside). The dotted lines mark the closed, zero current level. (b) Thermogram of K+binding to NaK2CNG-D in the presence of 150 mM NaCl (top). The integrated heat exchange from each injection is fit to a binding isotherm to obtain the relevant thermodynamic parameters (bottom). (c) Thermogram of Na+binding to NaK2CNG-D in the presence of 150 mM KCl. (d) The apparent affinity of K+ions for NaK2CNG-D as a function of NaCl concentration in solution. The line shows the fit to a competition binding equation described in the methods to obtainKD(K+) andKD(Na+); the mean of three or more experiments and their s.e.m. are plotted. Figure 3: Ion binding and permeation of NaK2CNG-D. ( a ) Single-channel traces at different membrane potentials (left) and the I – V curve (right). Currents are recorded with 150 mM NaCl+50 mM KCl in the cup (outside) and 200 mM KCl in the chamber (inside). The dotted lines mark the closed, zero current level. ( b ) Thermogram of K + binding to NaK2CNG-D in the presence of 150 mM NaCl (top). The integrated heat exchange from each injection is fit to a binding isotherm to obtain the relevant thermodynamic parameters (bottom). ( c ) Thermogram of Na + binding to NaK2CNG-D in the presence of 150 mM KCl. ( d ) The apparent affinity of K + ions for NaK2CNG-D as a function of NaCl concentration in solution. The line shows the fit to a competition binding equation described in the methods to obtain K D (K + ) and K D (Na + ); the mean of three or more experiments and their s.e.m. are plotted. Full size image To test the equilibrium ion selectivity of the NaK2CNG-D channel, we measured both Na + binding in the presence of competing K + ions and K + binding in the presence of competing Na + ions. As expected for a non-selective channel, we observed no measurable Na + binding in the presence of competing K + ions ( Fig. 3c ). However, we observed K + binding in the presence of Na + ions ( Fig. 3b ), which suggests that NaK2CNG-D is selective for K + at equilibrium; if the channel were non-selective, no heat from K + ion binding would have been observed, as the 150 mM Na + ions in the reaction chamber would outcompete the sub-millimolar K + ions injected from the syringe. The equilibrium selectivity of NaK2CNG-D for K + was quantified by measuring the apparent K + affinity as a function of Na + concentration as described for the NaK2K channel ( Fig. 3d ). A fit to the experimental data revealed a K + affinity of 28 μM and a Na + affinity of 11 mM ( Table 1 ). The fact that its individual ion-binding sites are so similar to those in K + channels likely explains the ~400-fold selectivity of the NaK2CNG-D channel for K + at equilibrium. Further support for this observation comes from the recent crystal structures of NaK2CNG-D channels determined at different ratios of Na + and K + ions. These structures show an increased K + occupancy in site 3 of the channel relative to the adjacent sites 2 and 4 in the presence of competing Na + ions (see companion paper) [32] . Therefore, site 3 of NaK2CNG-D is likely more K + -selective than the other two sites in the selectivity filter. Ion selectivity in the two-site NaK(D66N) channel Does further reducing the number of ion-binding sites alter the equilibrium selectivity? The two-site mutant NaK channel, D66N, has two of the canonical four ion-binding sites found in K + channels ( Fig. 1b ), but lacks the additional ion-binding sites found in the K + channels ( Fig. 1a ) [25] , [33] . We first determined the affinity and selectivity of this channel for K + and Na + at equilibrium using ITC. As with NaK2CNG-D, we observed no Na + binding to NaK (D66N) in the presence of high concentration of K + ions ( Fig. 4b ). In the presence of competing Na + ions, we observe K + binding demonstrating that NaK (D66N) is also selective for K + over Na + at equilibrium ( Fig. 4a ). By varying the concentration of Na + ions, the selectivity of this channel was determined to be 56 μM for K + and 18 mM for Na + giving an equilibrium selectivity of ~300 ( Fig. 4c and Table 1 ). Ion binding to NaK (D66N) has a Hill coefficient ( n ) of 1.0±0.1, suggesting a stoichiometric exchange of K + and Na + ions within the selectivity filter. 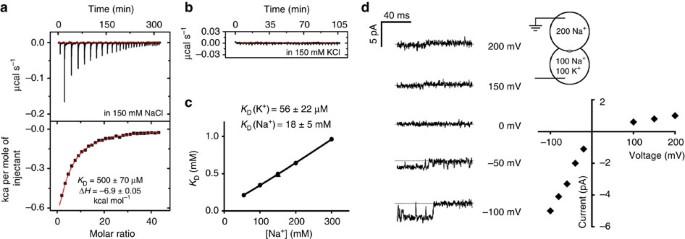Figure 4: Ion binding and permeation of NaK(D66N) channel. (a) Thermogram of K+binding to NaK(D66N) in the presence of 150 mM NaCl (top). The integrated heat exchange from each injection is fit to a binding isotherm to obtain the relevant thermodynamic parameters (bottom). (b) Thermogram of Na+binding to NaK(D66N) in the presence of 150 mM KCl. (c) The apparent affinity of K+ions for NaK(D66N) as a function of NaCl concentration in solution. The line shows the fit to a competition binding equation described in the methods to obtainKD(K+) andKD(Na+); the mean of three or more experiments and their s.e.m. are plotted. (d) Single-channel traces at different membrane potentials (left) and theI–Vcurve (right). Currents are recorded with 200 mM NaCl in the cup (outside) and 100 mM NaCl+100 mM KCl in the chamber (inside). The dotted lines mark the closed, zero current level. Figure 4: Ion binding and permeation of NaK(D66N) channel. ( a ) Thermogram of K + binding to NaK(D66N) in the presence of 150 mM NaCl (top). The integrated heat exchange from each injection is fit to a binding isotherm to obtain the relevant thermodynamic parameters (bottom). ( b ) Thermogram of Na + binding to NaK(D66N) in the presence of 150 mM KCl. ( c ) The apparent affinity of K + ions for NaK(D66N) as a function of NaCl concentration in solution. The line shows the fit to a competition binding equation described in the methods to obtain K D (K + ) and K D (Na + ); the mean of three or more experiments and their s.e.m. are plotted. ( d ) Single-channel traces at different membrane potentials (left) and the I – V curve (right). Currents are recorded with 200 mM NaCl in the cup (outside) and 100 mM NaCl+100 mM KCl in the chamber (inside). The dotted lines mark the closed, zero current level. Full size image We then determined the selectivity during ion conduction by measuring ion permeation using purified NaK (D66N) channels reconstituted into liposomes. Single-channel recordings using a vertical bilayer system were obtained with 200 mM NaCl on the outside and 100 mM KCl and 100 mM NaCl on the inside. These recordings show the channel conducts both K + and Na + ions, but Na + seems to conduct through the channel faster than K + ions ( Fig. 4d ). The membrane potential was varied from 200 to −100 mV to determine whether the channel is K + -selective based on its ion permeability ratio. In these conditions, a non-selective channel would reverse at zero millivolts and a K + -selective channel would reverse at a membrane potential much less than zero. As shown in Fig. 4d , NaK (D66N) is not K + -selective during conduction despite a strong K + selectivity at equilibrium. The small currents observed in K + or mixed Na + /K + limit our ability to determine whether NaK (D66N) is indeed non-selective, although both sides of the I – V curve could be seen as approaching 0 mV or a positive mV. NaK (D66N) shares the same two contiguous ion-binding sites as the wild-type non-selective NaK channel, suggesting that this channel is likely non-selective during ion conduction [22] . In this study, we asked whether the selectivity of a tetrameric cation channel is mirrored in its selectivity for binding ions at equilibrium. Our data show that K + -selective and non-selective channels select K + over Na + ions at equilibrium, demonstrating that equilibrium selectivity is insufficient to determine the selectivity of ion permeation. The preference for K + in both types of channels likely originates from their nearly identical individual ion-binding sites, which are known to bind K + ions better than Na + ions [34] , [35] . One fundamental difference between the non-selective and K + -selective channels is that the latter bind two or more K + ions, whereas the non-selective channels bind fewer ions in their filters. We hypothesize that although an equilibrium preference for K + is essential and is observed in all K + -selective channels, having multiple K + ions bound simultaneously is required for selective K + conduction in K + channels ( Fig. 5 ). 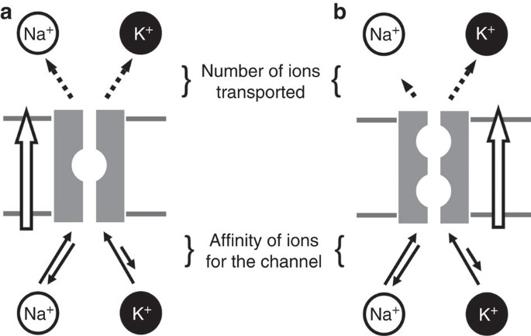Figure 5: Schematic summary of key observations. A representation of the (a) one ion- and (b) two ion-binding models for a channel. The circles within the channel represent the ion-binding sites. A membrane potential drives ions across the membrane from the inside to the outside (hollow arrows). Solid arrows indicate the rates of ion association and dissociation from the channel, which together determine the affinity (KD). The dashed arrows are proportional to the net number of ions that cross the membrane, the ratio of which determines the selectivity during ion conduction. Figure 5: Schematic summary of key observations. A representation of the ( a ) one ion- and ( b ) two ion-binding models for a channel. The circles within the channel represent the ion-binding sites. A membrane potential drives ions across the membrane from the inside to the outside (hollow arrows). Solid arrows indicate the rates of ion association and dissociation from the channel, which together determine the affinity ( K D ). The dashed arrows are proportional to the net number of ions that cross the membrane, the ratio of which determines the selectivity during ion conduction. Full size image What mechanism can explain the large equilibrium preference of NaK2CNG-D and NaK (D66N) channels for K + ions while displaying non-selective ion conduction? The model that is most consistent with the data presented here is that non-selective conductance of the NaK (D66N) channel arises from the similar rates at which Na + and K + bind, and the equal probability that a bound ion will dissociate on the other side of the membrane. If their concentrations are equal, then the probability that Na + and K + will bind the channel is determined by their k on rates; when the ion concentrations are different, the probability is determined by k on [X + ]. A small membrane potential will bias either ion to dissociate on one side of the membrane. The different k off rates for Na + and K + primarily alter how quickly an ion dissociates from the channel, not which side it will dissociate. So if the two ions have similar association rates and minimal barriers to ion transport, the conductance ratio will be the same as the ratio of ion binding and the channel would be non-selective for K + /Na + ions. The ion conduction selectivity of the NaK (D66N) channel can thus be explained simply by its high rate of conductance and the fact that it is occupied by a single ion at a time (the selective exclusion mechanism) [36] . The mechanism of K + -channel conduction selectivity is still under debate, but it is likely the result of both equilibrium and kinetic parameters [2] , [3] , [5] , [15] , [16] , [17] , [20] , [31] , [37] . The thermodynamic nature of the studies reported here prevents us from comparing these results directly to those of kinetic experiments. In addition, these ITC-based ion-binding experiments yield no information on the specific sites that the ions interact with in the selectivity filter or on the total number of ions bound in the filter. However, electrophysiology and crystallography experiments utilizing other K + channels show that at least two ions interact within the selectivity filter of K + channels during ion conduction, suggesting that two ions likely bind within the NaK2K channel [5] , [10] , [38] , [39] . An important difference between the non-selective and K + -selective mutant NaK channels is their number of ion-binding sites, which determines the number of ions that simultaneously occupy the channels during ion conduction. Multi-ion queues lead to the anomalous mole-fraction effect where the higher-affinity ions effectively block the conduction of lower-affinity ions [38] , [40] , [41] , [42] . This phenomenon allows the sites to equilibrate to their ion preference. In K + channels, K + ions would then primarily occupy the available sites in the filter, which leads to selective ion conduction under a variety of conditions [5] , [6] , [38] , [39] , [43] , [44] , [45] , [46] . We propose that the reduction in the number of K + ions bound in the two- and three-site channels effectively destroys the multi-ion selectivity mechanism utilized by K + channels. Three categories of K + transport systems (channels, transporters and carriers) likely achieve their selectivity against Na + by slowing down the transport process such that Na + is able to dissociate back into solution before ion transport takes place. In ion carriers, such as K + -selective nonactin or valinomycin, the time it takes to diffuse and enter the membrane is long enough to allow the ion-binding sites to equilibrate. In transporters, the requirement for a global conformational change slows transport rates to allow near-equilibration of the sites. The mechanism for K + channels is a multi-ion queue as discussed above. One possible evolutionary route from a K + transporter to a high-conductance K + channel is through mutations that allow a second K + ion to bind within the ion transport pathway. This simple process would retain selectivity although increasing the rate of conductance. By contrast, losing K + -binding sites without reducing the transport rate would lead to non-selective ion conduction. This is potentially the situation with the mutant KCNJ human K + channel that causes severe hypertension because of its loss of K + -selective ion-binding sites [47] . Protein expression and purification All mutant NaK channels are cloned into pQE60 expression vector without the first 19 amino acids. Plasmids were chemically transformed into M15[pREP4] Escherichia coli competent cells and grown overnight on LB agar plates containing 100 μg ml −1 ampicillin and 50 μg ml −1 kanamycin. The freshly grown colonies were used to inoculate LB media and the cultures grown at 37 °C to an OD 600 =0.8. Protein expression was induced with 0.4 mM IPTG (isopropyl β- D -1-thiogalactopyranoside) at 25 °C. Cells were harvested after 18 h of expression, spun down at 4,500 rpm using JA-10 rotor (Beckman Coulter) and stored at −80 °C. For purification, cells were re-suspended in 50 mM Tris buffer (pH 8.0), 150 mM KCl, 1 mM PMSF, 2 μg ml −1 DNase, 10 μg ml −1 lysozyme and 2 μg ml −1 leupeptin and lysed by sonication. n -Decyl-β- D -maltoside (DM) was added to the lysate to a final concentration of 40 mM and the mixture was incubated at room temperature for 3 h. The membrane-solubilized lysate was spun at 12,000 rpm in a JA-20 rotor (Beckman Coulter) for 20 min to clarify the solution. The supernatant was applied to Co 2+ resin (Clontech) equilibrated in 50 mM Tris (pH 8.0), 150 mM KCl, 5 mM DM, washed with buffer containing 15 mM imidazole and eluted in 300 mM imidazole. Thrombin was added to the elution (0.5 U mg −1 mutant NaK protein) and incubated for 5 h at room temperature to remove the His 6 tag. The digestion was stopped with 1 mM PMSF and the tetramer purified through a Superdex 200 (GE Healthcare) size exclusion column. Measuring ion-binding affinity using ITC Purified mutant NaK channels were concentrated to 25–150 μM depending on the enthalpy and affinity of each specific reaction. The protein was dialyzed against 50 mM Tris (pH 8.0), 50–400 mM NaCl, 5 mM DM immediately before use. ITC thermograms were collected on an iTC 200 (GE Healthcare) at 25 °C with a spinning speed of 1000, rpm. The sample chamber was filled with protein in the desired concentration of Na + and the injector syringe contained the same buffer with the addition of 5–60 mM KCl; the concentration of KCl was increased with higher NaCl concentrations as more K + was needed to saturate the channel. In the thermogram, the area under each downward deflection is the heat change of the system upon injecting a KCl solution into a chamber containing the channel. There are two primary sources of heat, the first is the heat of diluting the concentrated KCl solution into the chamber and the second is ion binding to the channel. The corresponding binding isotherm is generated from the integrated heat of each injection. The enthalpy ( H ) and apparent association constant ( K ) were fit in Origin (GE Healthcare) to a one-binding site model with the number of sites fixed to 1. The apparent dissociation constant K D (1/ K ) is reported in the text. As both Na + and K + ions compete within the channel’s selectivity filter, we determined the affinity of the empty channel for K + and Na + ions using the following competition equation: where is the fit apparent dissociation constant, and are dissociation constants for K + and Na + to the empty channel, and is a Hill coefficient. , and were fit using Prism (GraphPad Software). The equilibrium selectivity of the channel is the ratio / . Channel reconstitution and electrophysiology For reconstitution and electrophysiology, F92A was also mutated in the channels to increase their open probability [22] . A lipid mixture containing a 3:1 ratio of 1-palmitoyl-2-oleoyl-phosphatidylethanolamine (Avanti Polar Lipids) and 1-palmitoyl-2-oleoyl-phosphatidylglycerol (Avanti Polar Lipids) was dried and then re-suspended in reconstitution buffer containing 10 mM HEPES (pH 7.4), 450 mM KCl and 4 mM N-methyl- D -glucamine to a final concentration of 10 mg ml −1 . The lipid mixture were sonicated and solubilized in 10 mM DM for 1 h. Protein was added to a concentration of 0.1 mg protein per mg lipid with an additional 10 mM DM. The lipid-protein-detergent mixture was incubated overnight at room temperature before being dialyzed for 4–5 days to remove the detergent. Vesicles were flash frozen and stored at −80 °C. The activity of the NaK(D66N) channel was measured using a vertical lipid-bilayer set-up with 10 mM HEPES (pH 7.4), 1 mM EGTA and 200 mM NaCl in the cup (outside) and with 10 mM HEPES (pH 7.4), 1 mM EGTA, 100 mM NaCl and 100 mM KCl in the chamber (inside). The activity of NaK2K and NaK2CNG-D channels were measured with 200 mM KCl in the cup and 50 mM KCl and 150 mM NaCl in the chamber. Membrane voltage was controlled using a BC-535 Amplifier (Warner Instruments) with a Digidata 1440A analogue-to-digital converter (Molecular Devices). The currents were low-pass filtered at 1 kHz and were sampled at 20 kHz. Subsequent analyses were done using pClamp 10 (Molecular Devices). The lack of K + selectivity in NaK(D66N) was observed from three different channels in three independent experiments. The reversal potential for NaK2K was determined from six different channels, whereas the reversal potential for NaK2CNG-D was determined from three different channels. How to cite this article: Liu, S. & Lockless, S. W. Equilibrium selectivity alone does not create K + -selective ion conduction in K + channels. Nat. Commun. 4:2746 doi: 10.1038/ncomms3746 (2013).